Microwave transitions as a signature of coherent parity mixing effects in the Majorana-transmon qubit Solid-state Majorana fermions are generating intensive interest because of their unique properties and possible applications in fault tolerant quantum memory devices. Here we propose a method to detect signatures of Majorana fermions in hybrid devices by employing the sensitive apparatus of the superconducting charge-qubit architecture and its efficient coupling to microwave photons. In the charge and transmon regimes of this device, we find robust signatures of the underlying Majorana fermions that are, remarkably, not washed out by the smallness of the Majorana contribution to the Josephson current. It is predicted that at special gate bias points the photon-qubit coupling can be switched off via quantum interference, and in other points it is exponentially dependent on the control parameter E J / E C . We propose that this device could be used to manipulate the quantum state of the Majorana fermion and realize a tunable high coherence four-level system in the superconducting-circuit architecture. Photons are used to control and measure qubits in a diverse range of qubit systems from natural atoms to semiconducting and superconducting solid-state architectures [1] , [2] , [3] , [4] , [5] , [6] , [7] , [8] . The properties of solid-state qubits and resonators and coupling to photons can be engineered to some degree by design and this enables the combination of several different subsystems to form hybrid devices that take advantage of their relative strengths [9] , [10] . In turn, this leads to new methods of probing physical systems and, where highly quantum coherent subsystems are involved, to establishing control over their quantum variables. Of particular interest is the application of this approach to topological superconducting nanowires, as theoretical predictions [11] , [12] , [13] supported by experimental progress [14] , [15] indicate the presence of the highly sought-after Majorana zero-energy modes [16] , [17] localized on the wire around its end points. When the nanowire bridges a Josephson junction, the presence of Majorana zero modes was predicted to lead to several observable effects [18] , [19] , [20] , [21] , [22] , [23] , [24] , of which first experimental signatures were recently observed [25] and explained theoretically [26] . Even more intriguing is the case of an isolated mesoscopic Josephson junction, which in the absence of the nanowire is known as a Cooper–Pair–Box (CPB), embedded within an optical cavity. In addition to the Josephson coupling, charging effects and light-matter interactions play a pivotal role in this device. Using state of the art experimental progress the device can be engineered so that its charging energy is small compared with the Josephson energy, forming a highly coherent system known as the transmon [27] . When the nanowire is added, the presence of the Majorana zero modes modifies the properties of the device considerably; however, its high coherence should persist. The device can therefore be used as an alternative superconducting qubit. Its minimal quantum description involves two effective fermion degrees of freedom that arise from the Majorana zero modes and represent the parity state of the low-energy unpaired charges residing on the two sides of the Josephson junction. Similar set-ups were proposed as a basis for topological qubit construction [28] , [29] , [30] . Generically, the two fermions can couple and split through a Majorana coupling term generated by coherent single-electron tunnelling processes across the junction. In this likely relevant experimental scenario, a central question that needs to be addressed is what is the unique spectroscopic signature of the charge-neutral Majorana zero modes in such devices? In addition, can one establish control over the parity state, demonstrating its relevance for quantum information processing? To answer these questions, in this article we explore the microwave coupling in this device as compared with the traditional CPB. We discover a remarkable spectroscopic pattern consisting of two to four resonant frequencies whose number and intensities are tunable via a gate offset n g . This spectroscopic pattern is very different from the traditional transmon that admits exactly two resonant frequencies with non-tunable intensities. The excitation spectrum consists of multiple doublets inherited from the parity states. In the rest of this article we shall refer to the ground state doublet as the ‘Majorana-transmon (MT) qubit’. The combination of these properties allows: (i) spectroscopic detection of the parity state strengthening currently available transport signatures of Majorana fermions in a setting that avoids complications stemming from the need to attach leads and perform transport measurements, including weak antilocalization [14] , [31] , reflectionless tunnelling [32] and Kondo effects [33] ; and, (ii) coherent and tunable control over the parity state made possible by the highly anharmonic level structure and the tunability of transitions. As we demonstrate below, the coupling strengths for the different transitions are determined by a quantum interference of charge parities and reveal their presence. Such tunable control allows state manipulation of the MT qubit via the upper levels of what we will show to be a superconducting coherent double-Λ system. These properties are highly desirable for quantum-information processing in the superconducting qubit architecture, which is currently based on a very weakly anharmonic level structure that limits the speed and fidelity of gate operations. The source of weak anharmonicity, being the difference between adjacent transition frequencies, stems directly from the form and dominance of the Josephson energy in varieties of qubits that resist well to charge noise fluctuations [34] . Proposed set-up and description of the model The proposed hybrid device contains a nanowire that is placed in proximity to the Josephson junction of a CPB (see Fig. 1 ), the latter being a prototypical charge qubit (realized as either a two-dimensional (2D) or three-dimensional (3D) transmon). A combination of strong spin-orbit coupling and a Zeeman gap can be used to push the wire into its topological state, provided that the chemical potential is tuned within the wire’s gap. In this phase, Majorana zero modes with operators γ 2 and γ 3 are localized near the junction. Two additional distant Majorana modes are present within the superconductors, γ 1 and γ 4 (see Fig. 1 ). The operators satisfy and { γ i , γ j }= δ ij . The properties of the device are determined by the interplay of the Josephson coupling E J , the charging energy E C , the coupling E M between the Majorana excitations and the superconducting phase difference ϕ [18] , [20] , [35] , [36] , [37] , [38] , [39] , [40] . 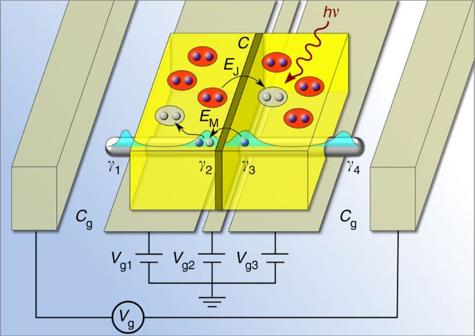Figure 1: The proposed experimental set-up. Two superconductors (yellow) form a Josephson junction and are capacitively coupled to control gates (grey). A topological nanowire (silver) lying in close proximity carries four Majorana zero modes. Two of the zero modes (green),γ2andγ3, hybridize across the junction, owing to coherent single-electron tunnelling processes, with strengthEM. The bottom gates control the density in the wire and the strength of the potential barrier between the two sides of the wire, tuning the value ofEM. The electrostatic offset charge,ng, is controlled via the side gates. The Hamiltonian for the hybrid junction is H = H T + H M where Figure 1: The proposed experimental set-up. Two superconductors (yellow) form a Josephson junction and are capacitively coupled to control gates (grey). A topological nanowire (silver) lying in close proximity carries four Majorana zero modes. Two of the zero modes (green), γ 2 and γ 3 , hybridize across the junction, owing to coherent single-electron tunnelling processes, with strength E M . The bottom gates control the density in the wire and the strength of the potential barrier between the two sides of the wire, tuning the value of E M . The electrostatic offset charge, n g , is controlled via the side gates. Full size image Here n g describes the total offset charge that represents an external electrostatic gate control. The anomalous term H M is generated by coherent single-electron tunnelling processes between the two superconductors facilitated by the overlap of the zero-energy Majorana modes across an electrostatic potential barrier. In our context, it allows coherent Rabi oscillations of unpaired electrons. We focus on the MT regime, which we define as E M ≪ E C ≪ E J , where the influence of charge noise is exponentially suppressed, and explore the dependence of the eigen state and eigen energy spectrum on n g . When E M is non-zero, we find a spectrum that is composed of closely spaced doublets of transmon-like energy levels, see Fig. 2 , with a periodicity of e compared with 2 e for the transmon. The microwave photons couple to the charge operator and we find that even when E M / E C ≪ 1 the charge matrix element that couples to the photon field is strongly dependent on n g and E J / E C for the allowed GHz-range transitions ( Fig. 2a ) since the bare states of the system become strongly hybridized. The MT level structure is highly anharmonic because of the fact that the third level is separated by an energy scale of the order of the plasma oscillation frequency that is much larger than the doublet level splitting ~ E M in the regime we consider. This could be traced back to the geometric origin where a nanowire with only a few channels would support a much smaller coupling E M compared with the macroscopic Josephson junction with E J , and the charging energy is controlled by the engineered capacitance. For completeness, we would like to mention other scenarios that were recently discussed in the literature: the E M =0 and E M = E C =0 limits in refs 28 , 29 ; the flux qubit in ref. 41 ; circuit QED extensions in refs 42 , 43 ; and, photon-induced long-distance Majorana coupling in ref. 44 . In contrast, the present work offers an effective model capturing the multilevel spectrum of the charge-qubit device. Owing to a particular set of useful features that we now elaborate on, this minimal scenario may also have considerable appeal as an alternative to transport-based experiments. 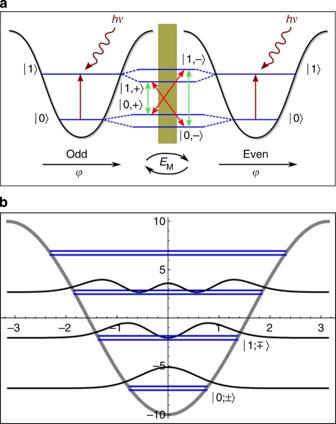Figure 2: The influence of coherent electron tunnelling between Majorana states on the transmon spectrum. (a) Schematic representative the bare eigenstates for the two parity states (depicted at the left and right potential wells) that are coherently mixed to form superposition states that constitute energy doublets (middle section). Tunable microwave couplings between the states (indicated by arrows) realize a double-Λ system. The various optical transition strengths can be controlled by varying eitherEJorng. (b) Representative probability densities of the two eigenstates denoted |0/1; ±› plotted against the background of the dominant Josephson energy potential, forEC/h=0.4 GHz,EJ/EC=25,EM/EC=5 × 10−4,ng=0.25. The doublet energy splittings are drawn exaggerated for visibility in the panels. Figure 2: The influence of coherent electron tunnelling between Majorana states on the transmon spectrum. ( a ) Schematic representative the bare eigenstates for the two parity states (depicted at the left and right potential wells) that are coherently mixed to form superposition states that constitute energy doublets (middle section). Tunable microwave couplings between the states (indicated by arrows) realize a double-Λ system. The various optical transition strengths can be controlled by varying either E J or n g . ( b ) Representative probability densities of the two eigenstates denoted |0/1; ±› plotted against the background of the dominant Josephson energy potential, for E C / h =0.4 GHz, E J / E C =25, E M / E C =5 × 10 −4 , n g =0.25. The doublet energy splittings are drawn exaggerated for visibility in the panels. Full size image Solution of the model In the topological phase and when E M =0, the nanowire excitations on each side of the potential barrier carry each a single zero energy fermion state, whose occupation becomes locked to the parity of the unpaired charge on the same side [35] , [38] , [45] , [46] , [47] , [48] . The parity of the total unpaired charge stays constant in the model and therefore the hamiltonian can be projected on two parity states that yields the form (see the Methods section for details) which we now diagonalize by solving the eigenvalue equation Hχ = Eχ where χ =( f ( ϕ ), g ( ϕ )) T . A crucial point is that one should take into account the requirement on the Hilbert space that f ( ϕ ) is periodic in ϕ with a periodicity 2 π , while g ( ϕ ) is antiperiodic. Alternatively, one can use a basis composed of solely periodic functions; however, the Hamiltonian gets modified according to H → H ′= U HU † , with U =diag{1, e i ϕ/2 } The eigen energies of this Hamiltonian were calculated numerically employing charge eigenstates and are presented in Fig. 3 as a function of n g . 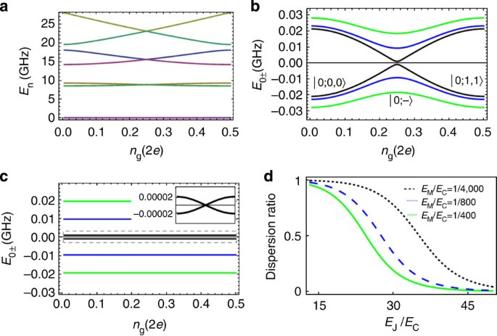Figure 3: Calculated spectra of the full Hamiltonian for different parameter regimes. (a) Spectrum of the Majorana-Cooper-Pair-Box spectrum withEJ/h=10 GHz,EC/h=0.4 GHz forEJ/EC=25 andEM/EC=1/400 as a function of the charge offsetng. An avoided crossing of orderEMdevelops (b) between the states of different parity and the periodicity of the spectrum is halved, to repeat whenng→ng+1/2. The ground state pair is shown forEM/EC=1/1,400 (black),EM/EC=1/140 (blue) andEM/EC=1/70 (green) forEJ/EC=7.14 (withEC/h=1.4 GHz). (c) ForEJ/EC=25 the parity states forEM=0 are crossing but exponentially close in energy with a dispersion of ε0+(EM=0)/h=2 × 10−5GHz (see inset graph of the grey dashed area, with samexaxis). However, including the Majorana coupling,EM>0 effectively removes the degeneracy and determines the energy splitting in the whole range ofng. (d) In the transmon regime the residual dispersion is further suppressed by the Majorana interactionHM, as the plot of dispersion ratioε1+(EM)/ε1+(0) shows. Figure 3: Calculated spectra of the full Hamiltonian for different parameter regimes. ( a ) Spectrum of the Majorana-Cooper-Pair-Box spectrum with E J / h =10 GHz, E C / h =0.4 GHz for E J / E C =25 and E M / E C =1/400 as a function of the charge offset n g . An avoided crossing of order E M develops ( b ) between the states of different parity and the periodicity of the spectrum is halved, to repeat when n g → n g +1/2. The ground state pair is shown for E M / E C =1/1,400 (black), E M / E C =1/140 (blue) and E M / E C =1/70 (green) for E J / E C =7.14 (with E C / h =1.4 GHz). ( c ) For E J / E C =25 the parity states for E M =0 are crossing but exponentially close in energy with a dispersion of ε 0+ ( E M =0)/ h =2 × 10 −5 GHz (see inset graph of the grey dashed area, with same x axis). However, including the Majorana coupling, E M >0 effectively removes the degeneracy and determines the energy splitting in the whole range of n g . ( d ) In the transmon regime the residual dispersion is further suppressed by the Majorana interaction H M , as the plot of dispersion ratio ε 1+ ( E M )/ ε 1+ (0) shows. Full size image Further insight into the effect of the coupling H M on the system can be gained from diagonalizing the Hamiltonian in the basis of the transmon eigenfunctions [34] that will be denoted as Ψ k ( n g , ϕ ) and which diagonalize H T [ n g ] and H T [ n g +1/2], respectively. In this basis, H ′ can be shown to be approximately 2 × 2 block diagonal since H M mostly couples the same band pairs {Ψ k ( n g , ϕ ), Ψ k ( n g +1/2, ϕ )}. This coupling results in an energy splitting of the order E M developing around n g =1/4 (see Fig. 3b) ) while further from this point it is a function of both E M and the dispersion (which is defined as the amplitude of the variation of a specific eigenenergy with respect to n g ). Importantly, the periodicity of the energy levels is halved, and this will affect the behaviour of the system with respect to tunnelling of non-equilibrium quasiparticles. Further, in the transmon regime E J / E C >>1 the dispersion of the transmon levels is exponentially suppressed such that the E M dominates the spectral gap and flattens it further, see Fig. 3c,d , and hence improving its famous resilience against dephasing caused by charge fluctuations. Each energy eigenstate can be described as pseudospin in the two-dimensional state space of unmixed parities associated with the one transmon band states of H T [ n g ] and H T [ n g +1/2]. We denote these by | k ,±›=( f k , , g k, ) T where k =0, 1, … denotes the transmon band index and ± denotes the amplitude pairs that become exactly symmetric and antisymmetric at the degeneracy point n g =1/4. In the vicinity of this point, interaction H M strongly correlates the parity and phase ( ϕ ) with close-to-equal weight hybridization, that is, | f 2 |−| g 2 |=0 (‹ σ Z ›=0). The resulting pseudospin nature of the wave function can be depicted by taking the partial trace in the pseudospin space , see Fig. 4a . The ϕ -dependent pseudospin lies on the equator of the Bloch sphere because of the equal weighting. It points predominantly in the σ x direction since the parity of the transmon wave functions with respect to ϕ yields real matrix elements for H M . 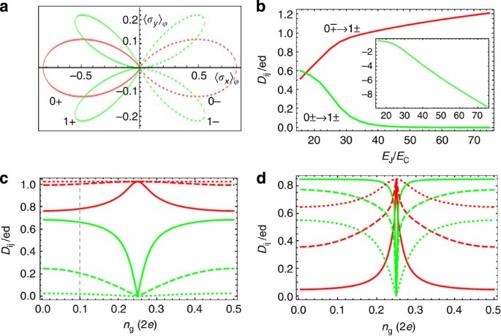Figure 4: Phase-parity-correlated states and their optical coupling. (a) The fermion tunnelling termHMleads to a correlation between the superconducting phase difference (ϕ) and the parity pseudospin. Thex–yprojection of the Bloch vector representation of the parity pseudospin is plotted as a function ofϕat the point of maximal hybridizationng=1/4. (b) Dependence of the optical transition strengthk,s→k′,s′as function ofEJ/ECwithEC/h=0.4 GHz,ng=0.1 andEM/EC=1/400, and the logarithm of this dependence (inset, samexaxis) shows that the suppression is exponential. (c) Dependence of the dipole on the effective gate chargengforEJ/EC=40 withEC/h=0.4 GHz, and forEJ/EC=20 (d). Three curves are drawn in each panel (c,d) to show the dependence onEM/EC=2.5 × 10−3(dotted), 2.5 × 10−4(dashed), 2.5 × 10−5(solid). Strong parity-phase correlations arise near the avoided crossing pointng=1/4 which result in a vanishing of the coupling between the |0→1; ±› states. Deeper in the transmon regime (EJ/EC=40) these correlations persist across the whole range ofngeven for small values of the Majorana couplingEMthat suppresses the optical coupling matrix element, see dotted line inc. Figure 4: Phase-parity-correlated states and their optical coupling. ( a ) The fermion tunnelling term H M leads to a correlation between the superconducting phase difference ( ϕ ) and the parity pseudospin. The x – y projection of the Bloch vector representation of the parity pseudospin is plotted as a function of ϕ at the point of maximal hybridization n g =1/4. ( b ) Dependence of the optical transition strength k,s → k′,s ′ as function of E J / E C with E C / h =0.4 GHz, n g =0.1 and E M / E C =1/400, and the logarithm of this dependence (inset, same x axis) shows that the suppression is exponential. ( c ) Dependence of the dipole on the effective gate charge n g for E J / E C =40 with E C / h =0.4 GHz, and for E J / E C =20 ( d ). Three curves are drawn in each panel ( c , d ) to show the dependence on E M / E C =2.5 × 10 −3 (dotted), 2.5 × 10 −4 (dashed), 2.5 × 10 −5 (solid). Strong parity-phase correlations arise near the avoided crossing point n g =1/4 which result in a vanishing of the coupling between the |0→1; ±› states. Deeper in the transmon regime ( E J / E C =40) these correlations persist across the whole range of n g even for small values of the Majorana coupling E M that suppresses the optical coupling matrix element, see dotted line in c . Full size image Light–matter interaction Electromagnetic fields influence the dynamics of the MT by coupling via the dipole operator, given by D = ide ∂ ϕ , where d is the distance between the two superconductors. In the transformed basis, D ′= U DU † the dipole operator acquires the form The parity-phase correlation has important consequences for the microwave and RF coupling between the states. The matrix elements of the dipole operator where s , s ′=±, yield the coherent sum of two matrix elements resulting from the different fermion parities. Thus, the transition amplitude between states of same or different s , s ′ is given by the coherent addition of the matrix elements (see Fig. 2a ). Usually, the integrals need to be evaluated numerically; however, some observations can be made on general grounds. At the degeneracy point, n g =1/4 the parity pseudospin state amplitudes have equal weight of uncoupled MT components and the matrix elements for the transitions |0; s ›→|1; s ′› become where the relative sign ± depends on the choice of pair of states. As we show in the Methods section for the transitions corresponding to |0; ±›→|1; ±› there is a full destructive interference between the dipole matrix elements at n g =1/4. As we move away from the special point n g =1/4, the amplitudes change and the dipole coupling returns to a finite value on a scale that depends on E M , see Fig. 4 . In contrast, the ‘intraband’ dipole coupling k,s → k,s ′ can be shown to be relatively small for all values of n g . Detectible experimental signatures As n g is varied, it should be possible to see the number of transition lines indicated in Fig. 2a change. A spectroscopic pattern ( Fig. 5 ) that is essentially different from the one of the transmon would emerge. It arises from the excitation spectrum that consists of multiple doublets inherited from the charge parity states (see Fig. 2b ). A dominant feature in the pattern is that the strength of the parity-conserving transitions (green), see Fig 2a , can be tuned to exactly zero by the gate offset n g or exponentially suppressed by varying the ratio E J / E C ( Fig. 4b–d ). The former appears as a hole in the middle of the spectrum (see Fig. 5 ). This pattern depends on the Majorana coupling E M and the latter may be estimated from it. In the following paragraph we show that this pattern is robust against additional residual interactions such as γ 1 γ 2 , γ 1 γ 4 and γ 3 γ 4 couplings or when several transverse modes exist in the wire. A sensitive experimental technique [49] that relies on the Ramsey measurement was used recently for temporally tracking minute changes in the spectrum of the transmon (of the order of %0.04 of the transition frequency). It was demonstrated that for a device that has similar parameters to the one discussed here the transition rate for non-equilibrium quasiparticles was slow enough (milliseconds regime) to allow temporal tracking of the spectral structure. From our model analysis it arises that if combined with bias gates that influence n g and the strength of the coherent tunnelling process E M , such demonstrated experimental sensitivity would be arguably be sufficient for (1) detecting the additional transition frequencies in the transmon regime E J / E C >>1, (2) achieving, in a split CPB configuration, a strong on–off control of the coupling to microwave photons, see Fig. 4b . In a split CPB configuration of the transmon device it is possible to control the effective Josephson energy E J by varying the external flux through the loop [34] . In the hybrid MT model the sensitivity of the dipole coupling to parameters also extends to an exponential dependence on the ratio of E J / E C since the latter controls the relative effectiveness of the hybridization created by H M , and (3) detecting the disappearance of two spectral lines exactly at the degeneracy point n g =1/4. Other methods of strongly controlling the coupling were designed and demonstrated recently [50] , [51] , [52] using a split CPB strongly coupled to a cavity, albeit with a qualitatively different behaviour since the dependence on E J / E C requires precise tuning to one point in order to turn off the coupling. 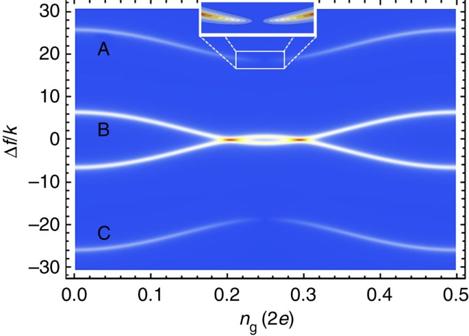Figure 5: Predicted spectroscopy of a Majorana-transmon qubit device. The microwave transition frequencies (Δf) of the system as function of the offset chargengfor the different transition paths within the lower part of the spectrum. Away fromng=1/4, the upper (A) and lower (C) lines are associated with the usual transmon transitions, while the central lines (B) describe parity-mixing effects and are a unique feature of the Majorana modes. In addition, atng=1/4 the transition amplitudes in each parity manifold interfere destructively and this gives rise to another unique feature, a ‘spectral hole’ in transition (A, C). In contrast to the traditional transmon, all spectral lines are gate-tunable, and the pattern can be shifted between four (left) and two (centre) resonant frequencies. The frequencies are plotted relative to the average and in units of the line widthκ/2π=50 KHz, takingEC/2π=400 MHz,EJ/EC=27 andEM/2π=0.5 MHz. Figure 5: Predicted spectroscopy of a Majorana-transmon qubit device. The microwave transition frequencies (Δ f ) of the system as function of the offset charge n g for the different transition paths within the lower part of the spectrum. Away from n g =1/4, the upper (A) and lower (C) lines are associated with the usual transmon transitions, while the central lines (B) describe parity-mixing effects and are a unique feature of the Majorana modes. In addition, at n g =1/4 the transition amplitudes in each parity manifold interfere destructively and this gives rise to another unique feature, a ‘spectral hole’ in transition (A, C). In contrast to the traditional transmon, all spectral lines are gate-tunable, and the pattern can be shifted between four (left) and two (centre) resonant frequencies. The frequencies are plotted relative to the average and in units of the line width κ /2 π =50 KHz, taking E C /2 π =400 MHz, E J / E C =27 and E M /2 π =0.5 MHz. Full size image Finite size effects and multimode wire In the following, we discuss two central mechanisms that may modify the spectroscopic spectrum of the MT device. The first mechanism is related to the appearance of additional Majorana couplings, as can result from the finite size of the wire or from certain disorder effects. The second mechanism results from the presence of additional transverse modes in the wire interacting via the charging energy. As we now argue, the rich spectroscopic interference patterns that occur in these cases display very similar characteristics compared with the pure case discussed before, demonstrating a certain robustness of these results. First, we consider the case that additional Majorana couplings exist, such that H M is replaced by Introducing fermions via and , as described in the Methods section, and projecting on their occupations |00› and |11› (constraining our discussion to the even subspace, without loss of generality), we get the modified Hamiltonian where λ =( λ 12 + λ 34 )/2 and E M =( λ 23 + λ 14 )/2. This results in the introduction of a new energy scale λ that repels the Transmon energies associated with the uncoupled states |00› and |11›. For the case λ >> E M , by tuning now the Transmon dispersion, one can reach the limit that the coupling energy E M will become ineffective. This leads to exponential sensitivity to the presence of λ >> E M that can further help to differentiate higher energy spurious states from the zero mode states. For the Majorana modes we expect on physical grounds that the coupling strengths satisfy λ ≪ E M . The resulting spectroscopic pattern is displayed for several values of λ ≤ E M in Fig. 6 , using the same parameters as in Fig. 5 . 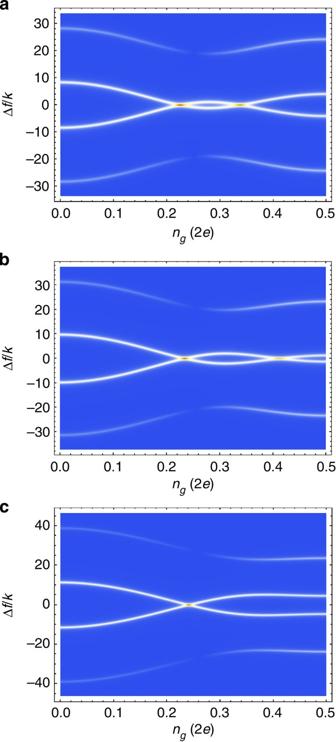Figure 6: Spectroscopic signatures in the presence of additional Majorana couplings for different coupling strengths. The spectral holes aroundng=1/4 for the outer spectroscopic lines are unaffected by the coupling strengthλ. Asλgets closer in size toEM, one of the spectral nodes in the centre of the pattern coalesces with its mirror image. At even larger values ofλ, the two outer spectral lines quickly lose weight. The pattern demonstrates a periodicity inngwith a double period 2e, while the halved periodicity is lost because of the presence of the additional couplings shifting all Majorana zero modes away from zero energy. (a)λ=EM/4, (b)λ=EM/2 and (c)λ=EM. Figure 6: Spectroscopic signatures in the presence of additional Majorana couplings for different coupling strengths. The spectral holes around n g =1/4 for the outer spectroscopic lines are unaffected by the coupling strength λ . As λ gets closer in size to E M , one of the spectral nodes in the centre of the pattern coalesces with its mirror image. At even larger values of λ , the two outer spectral lines quickly lose weight. The pattern demonstrates a periodicity in n g with a double period 2 e , while the halved periodicity is lost because of the presence of the additional couplings shifting all Majorana zero modes away from zero energy. ( a ) λ = E M /4, ( b ) λ = E M /2 and ( c ) λ = E M . Full size image Next, we consider the case that there are two transverse modes in the wire (one can also extend straightforwardly the analysis to additional transverse modes). Consequently, one should double all Majorana zero modes and obtain two sets γ i and where i =1,…,4. The modified H M is We stress that the problem is not trivially doubled owing to the presence of a charging energy, which is only sensitive to the total unpaired charge. We introduce additional fermions and . Using the notation for the occupations of the fermions, the full charge basis is |00; 00› e iℓ ϕ , |01; 01› e im ϕ , |10; 10› e ip ϕ and |11; 11› e iq ϕ , where ℓ , q εZ and m , p εZ+1/2. The full Hamiltonian can be written in this basis as where the matrices σ i ⊗ τ j are composed of two copies of Pauli matrices. We present the resulting spectroscopic pattern in Fig. 7 using the same parameters as in Fig. 5 and for several values of . The resulting spectroscopic pattern looks like two copies of the single-mode spectrum, shifted up and down by . Although more complex interference effects occur when , the two outer lines remain well decoupled from their respective other copy, and the spectral hole in the two outer lines consequently persists. 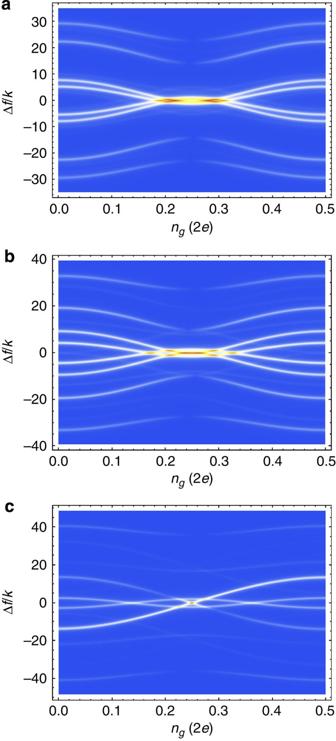Figure 7: Spectroscopic signatures of the two-mode wire as function of the second mode coupling. As the second mode (with coupling strengthE′M) is turned on, the spectrum initially behaves like two shifted copies of the single-mode spectrum. Whengets larger, more complex interference patterns appear. However, it can be seen that the spectral holes aroundng=1/4 for the outer spectroscopic lines remain robust across the transition from one mode to two modes, albeit their overall visibility noticeably decreases. (a)E′M=EM/4, (b)E′M=EM/2 and (c)E′M=EM. Figure 7: Spectroscopic signatures of the two-mode wire as function of the second mode coupling. As the second mode (with coupling strength E ′ M ) is turned on, the spectrum initially behaves like two shifted copies of the single-mode spectrum. When gets larger, more complex interference patterns appear. However, it can be seen that the spectral holes around n g =1/4 for the outer spectroscopic lines remain robust across the transition from one mode to two modes, albeit their overall visibility noticeably decreases. ( a ) E ′ M = E M /4, ( b ) E ′ M = E M /2 and ( c ) E ′ M = E M . Full size image A device that realizes this Hamiltonian could have substantial advantages over current superconducting qubit devices: (1) in addition to the gate tunability of the direct microwave coupling between transmon qubit states, the two lowest MT states form an energy doublet, see Fig. 2 , which constitutes a highly anharmonic MT qubit. The high anharmonicity is considered a benefit for qubit state manipulation as it reduces the probability of higher states being excited and shortens the duration of control pulses. (2) The two almost degenerate ground states can be regarded as part of a Λ type system and thus optically manipulated via transitions involving the higher doublet states. (3) The sensitivity of the states to the parameter n g leads to adiabatic control, which by tuning n g from 0 to 1/2 will take a system prepared, for example, in a state pointing predominantly in the | k ; 0, 0› direction to a state close to | k ; 1, 1›. Microscopically, a Cooper pair is split coherently and adiabatically between the two sides of the junction generating the transition between the two parity states. Microscopic two-level systems (TLS) that interact with the charge qubit generally give rise to spurious spectroscopic signatures. However, these can be differentiated from the case of Majorana fermions. In the case of a TLS that is resonantly coupled to the transmon there is only one ground state and therefore only two spectroscopic transitions to the one-excitation manifold. Correspondingly, there are only two transition frequencies that can be observed compared with up to four in the Majorana case. In contrast, if the TLS is close to degenerate in energy, the full system may possess a similar spectrum of two doublets. However, the crucial difference arises from the absence of direct coupling between the two quasi-degenerate ground states, in contrast to the case of Majorana fermions. This strongly suppresses any additional features in the spectroscopic pattern. Another possible scenario is a single electron state trapped within the oxide barrier, with a typical energy E 0 , that can exchange electrons with the two superconductors. Again, the phenomenology is very different since there will always be an extra energetic cost associated with an unpaired electron within the superconductors, leading to a very high energy scale E 0 +Δ in which such processes appear in the spectroscopic pattern (here Δ is the superconductor gap). Generally speaking, independently of the competing microscopic scenario, as long as zero energy Majorana modes exist in the sample: (i) the periodicity of the spectrum is coherently halved compared with the regular transmon owing to a rigidity in the relative shift n g → n g +1/2 of the two levels that hybridize to form the doublet; and, (ii) the spectroscopic signatures do not depend on the particular realization of randomly occurring TLSs in the oxide. Finally, semiconductor nanowires would probably contain a certain degree of disorder. Qualitatively, if the disorder is long ranged and smooth on the scale of the lattice constant, it could effectively act as a random potential that fragments the nanowires into sections of topologically trivial and non-trivial phases. Within the theoretical framework of topological superconductrors, this would cause the appearance of additional Majorana pairs along the nanowire. However, only couplings between Majorana zero modes residing on opposite sides of the Josephson junction would couple to the superconducting phase difference and hence to the photons. In contrast, the rest of the Majorana zero modes would be passive spectators in this process and hence we do not expect the signatures described here to disappear. Derivation of the Hamiltonian The mesoscopic nature of the Majorana-CPB prescribes certain intricacies in the diagonalization procedure that we now elaborate on. It is a common practice to compose non-local Dirac fermion zero modes , and similarly , through hermitian conjugation. This choice of basis simplifies the calculations as well as the presentation of our solution. By doing so we retain vital information regarding the different boundary conditions for the even and odd sectors of the charge transfer operator. This is also compatible with our goal of calculating the dipole matrix elements, which is very naturally written as a diagonal operator in our basis. This set of operators satisfies the canonical anticommutation relations for fermions, . In addition, we introduce a number operator for each superconductor that we denote by which counts the number of Cooper pairs in units of 1, and which is conjugate to the superconducting phase, . Importantly, in topological superconductors can assume both integer and half-integer eigenvalues. The latter are associated with the presence of an unpaired electron, counted as half a Cooper pair. We initialize the system by considering, in the absence of tunnelling across the junction, a definite parity of the electron number within each superconductor. The occupation of the Dirac zero mode is thus set by the parity of the electron number, N i =2 n i (mod 2). Let us denote the initial state of the two Dirac zero modes within one doublet by | N 1 , N 2 ›. For simplicity we also assume that initially n 1 = n 2 (different choices lead to slightly different formulations but the physical results remain the same up to an overall shift of the gate charge). Next we turn on the couplings E M and E J associated with single-electron tunnelling and Cooper-pair tunnelling, respectively. We construct basis states for the even and odd parity sectors and relative number of Cooper pairs where and ϕ = ϕ 1 − ϕ 2 is the relative phase satisfying . The first (second) set of wave functions is periodic (antiperiodic) under a change of ϕ by 2 π . The Cooper-pair tunnelling operator modifies the eigenvalue of by ±1, hence only couples states internally within the two subspaces (9) and (10). In contrast, the single-electron tunnelling operator intermixes the two subspaces. To model the latter we introduce electron raising and lowering operators satisfying . These operators are double-valued as they change sign when ϕ i → ϕ i +2 π and need to be matched with the Majorana zero mode operator that also changes sign, leading to admissible operators (the spectrum is necessarily 2 π periodic, although some parity constrained states may exhibit 4 π periodicity). The single electron tunnelling term is thus written in terms of the relative phase and the Majorana zero modes as in Equation (1), with fully shuffling the state of the zero mode occupations: . In addition, the phase-dependent part of the electron tunnelling operator ensures that the eigenvalue of changes by ±1/2. Hence, states of the form (9) can only couple to states of the form (10). By projecting on the orthogonal states | N 1 , N 2 › and the Hamiltonian acquires a matrix structure, see Equation (2), or in the alternative basis, Equation (3). Coherent interference On the basis of Equation (B3) in ref. 34 it can be shown that the characteristic values ν of the Mathieu functions in the transmon wave functions obey . From this, it is straightforward to show that the transmon wave functions obey based on the symmetry properties for non-integer Mathieu functions with respect to ν . The degeneracy point n g =1/4 is special since it obeys n g +1/2=1− n g from which it follows that and therefore the expression for the dipole can be written solely in terms of wave functions at n g =1/4. Employing in addition on the symmetry properties for non-integer Mathieu functions with respect to the phase ϕ it follows that for the transitions corresponding to |0; ±›→|1; ±› there is a full destructive interference between the dipole matrix elements. How to cite this article : Ginossar, E. and Grosfeld, E. Microwave transitions as a signature of coherent parity mixing effects in the Majorana-transmon qubit. Nat. Commun. 5:4772 doi: 10.1038/ncomms5772 (2014).